Dynamic GATA4 enhancers shape the chromatin landscape central to heart development and disease How stage-specific enhancer dynamics modulate gene expression patterns essential for organ development, homeostasis and disease is not well understood. Here, we addressed this question by mapping chromatin occupancy of GATA4—a master cardiac transcription factor—in heart development and disease. We find that GATA4 binds and participates in establishing active chromatin regions by stimulating H3K27ac deposition, which facilitates GATA4-driven gene expression. GATA4 chromatin occupancy changes markedly between fetal and adult heart, with a limited binding sites overlap. Cardiac stress restored GATA4 occupancy to a subset of fetal sites, but many stress-associated GATA4 binding sites localized to loci not occupied by GATA4 during normal heart development. Collectively, our data show that dynamic, context-specific transcription factors occupancy underlies stage-specific events in development, homeostasis and disease. Transcription factors (TFs) drive spatiotemporal patterns of gene expression that control the development of organs and their responses to disease. How TFs are redeployed to regulate distinct stage-specific gene expression programs is not well understood. A fundamental step towards answering this question is to delineate dynamic changes in TF occupancy and chromatin context in development and disease. Development of the heart is orchestrated by a set of cardiac TFs. In adult heart disease, many of the same TFs regulate the heart’s stress responses [1] . Indeed, many fetally expressed genes are re-expressed in adult heart disease, and this has been interpreted as disease-induced reactivation of a fetal transcriptional programme. To gain insights into how cardiac TF activity is regulated to drive stage-specific transcriptional programme, we studied the master cardiac TF GATA4, which is required in the heart from cardiomyocyte specification through adulthood [2] , [3] , [4] , [5] , [6] , [7] . Using a knock-in allele of GATA4 that is biotinylated in vivo to permit high-affinity GATA4 pulldown [8] , we mapped the changes in GATA4 chromatin occupancy that occur between fetal versus adult heart. GATA4 bound to loci with active chromatin signatures, and indeed GATA4 contributed to establishing this active chromatin signature by stimulating H3K27ac deposition, which facilitated GATA4-driven gene activation. Furthermore, our data revealed that some GATA4 binding sites are maintained between fetal and adult heart, but that most change dynamically between developmental stages. GATA4 occupancy studies of control versus pressure overloaded adult heart similarly showed that some fetal GATA4-bound regions were restored in cardiac hypertrophy, but most hypertrophy-induced GATA4 regions were newly established elements of an adult hypertrophic transcriptional programme. Identification of GATA4 regulated enhancers in fetal heart We previously reported an allele of GATA4 in which the endogenous gene has been modified to incorporate FLAG and bio (flbio) epitope tags [8] , [9] , where bio is a 23 amino-acid sequence specifically biotinylated by the enzyme BirA [10] . In GATA4 flbio/flbio ::Rosa26 BirA/+ mice, GATA4 flbio is pulled down with high affinity onto immobilized streptavidin. The GATA4 flbio allele retains full or nearly full activity [11] . Using this high-affinity system, we identified GATA4 peaks in E12.5 heart ventricles by bioChIP-seq. In each of the two biological duplicate samples, we identified over 50,000 GATA4-bound regions (hereafter referred to as GATA4 regions), with 43,800 (85.0%) shared between the duplicates ( Fig. 1a ; Supplementary Data 1 ). Around 50.8% of these regions overlapped with GATA4 flbio binding sites in HL1 cardiomyocyte-like cells [8] . We also performed GATA4 antibody-based chromatin immunoprecipitation (ChIP)-seq and found that it was less sensitive, identifying 11,915 (72.7%) regions that were shared between biological duplicates ( Fig. 1a ). Around 11,561 of these regions (97%) were also enriched by the GATA4 bioChIP-seq. We refer to these peaks shared between all four samples as high confidence fetal GATA4 regions. 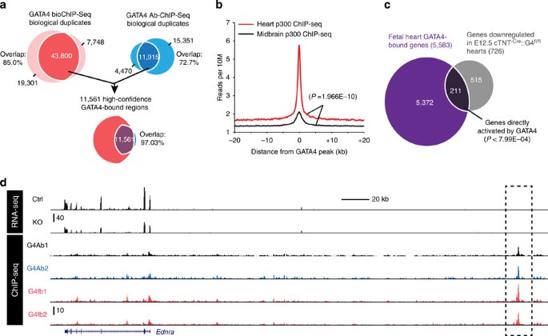Figure 1: GATA4 regulates genes expression through GATA4-bound enhancers during embryonic heart development. (a) Identification of GATA4 peaks in embryonic E12.5 heart through GATA4 bioChIP-seq and GATA4 antibody-based ChIP-seq. (b) p300 ChIP-seq reads13from heart and midbrain near GATA4 peaks in embryonic heart. There was significantly greater enrichment of heart p300 signal near GATA4 peaks compared with brain p300 signal. (Kolmogorov–Smirnov test). (c) Overlapping of GATA4 enriched genes with genes downregulated in E12.5 cTNT-Cre::G4fl/flembryonic heart. Gene expression was measured by RNA-seq. (d) Visualization of GATA4 ChIP-seq and RNA-seq data tracks. G4fb, bio-tagged GATA4-based ChIP-seq; G4Ab, GATA4 antibody-based ChIP-seq. Dashed box indicates a distal high confidence GATA4 region associated withEdnra. Figure 1: GATA4 regulates genes expression through GATA4-bound enhancers during embryonic heart development. ( a ) Identification of GATA4 peaks in embryonic E12.5 heart through GATA4 bioChIP-seq and GATA4 antibody-based ChIP-seq. ( b ) p300 ChIP-seq reads [13] from heart and midbrain near GATA4 peaks in embryonic heart. There was significantly greater enrichment of heart p300 signal near GATA4 peaks compared with brain p300 signal. (Kolmogorov–Smirnov test). ( c ) Overlapping of GATA4 enriched genes with genes downregulated in E12.5 cTNT-Cre::G4 fl/fl embryonic heart. Gene expression was measured by RNA-seq. ( d ) Visualization of GATA4 ChIP-seq and RNA-seq data tracks. G4fb, bio-tagged GATA4-based ChIP-seq; G4Ab, GATA4 antibody-based ChIP-seq. Dashed box indicates a distal high confidence GATA4 region associated with Ednra . Full size image GATA4 interacts with the transcriptional co-activator and histone acetyltransferase p300 (ref. 12 ), and GATA4 enhances p300 recruitment to chromatin loci [8] . Therefore, we asked if heart p300 binding sites [13] were overrepresented near high confidence fetal heart GATA4 peaks ( Fig. 1b ). Indeed, heart p300 ChIP-seq reads were strongly enriched on GATA4 peaks, but midbrain p300 ChIP-seq reads were not ( Fig. 1b ; P =2.0E−10). Because the fetal p300-bound regions were predictive of fetal heart enhancer activity [13] , these data indicate that GATA4 regions contain functional transcriptional enhancers. These data extend this work to provide unbiased, genome-wide support for GATA4 recruitment of p300 to heart enhancers. Identifying genes directly activated by GATA4 We used RNA-seq on E12.5 cTNT-Cre::Gata4 fl/fl (G4 CKO ) and control heart ventricles to identify genes regulated downstream of GATA4. There were 1,720 differentially expressed genes (log 2 fold change >0.5). GATA4 promoted expression of 726 genes (that is, downregulated in loss of GATA4), and 211 of them were associated with one or more GATA4 regions ( P <7.99E−04) ( Fig. 1c and Supplementary Data 2 ). These 211 genes are likely to be directly activated by GATA4, and their 511 associated GATA4 regions are candidate GATA4-dependent enhancers. The 211 genes were overrepresented for gene ontology (GO) terms linked to heart and muscle development ( Supplementary Fig. 1a ). One example is Ednra , encoding an endothelin receptor, which was downregulated twofold in GATA4 loss-of-function and was linked to a strong GATA4 region 264 kb upstream of the transcriptional start site (TSS; Fig. 1d ) as well as two additional intergenic peaks downstream of Ednra (not shown). In addition, 422 genes that were bound by GATA4 and upregulated in G4 CKO heart ventricles ( Supplementary Fig. 1b ), suggestive of direct GATA4-mediated repression. These 422 genes were overrepresented for genes with functional annotations related to heart and vasculature development ( Supplementary Fig. 1c ). To evaluate the prediction that GATA4 regions linked to the 211 GATA4-activated genes are functional transcriptional enhancers, we tested 12 candidates linked to 4 genes ( Ednra , Hey2 , Kcne1 and Hopx ) in transient transgenic enhancer assays. Around 7 of these 12 enhancers (58.3%) were active in the heart ( Table 1 ; Fig. 2a and Supplementary Fig. 2 ), although the activity of one of these, Hey2 –8, was confined to non-cardiomyocytes of the outflow tract cushion. We previously tested putative enhancers based on multiple transcription factor occupancy in cardiomyocyte-like HL1 cells, and one of these tested enhancers met the criteria used to select enhancers for this study [8] . This enhancer also exhibited strong heart transcriptional activity. Overall, a GATA4 region linked to gene downregulation in G4 CKO predicted heart enhancer activity (8/13, 61.5%), comparable to the frequency of p300-bound regions with heart enhancer activity (62.3%, ref. 14 ). The highest frequency of heart enhancer activity occurred for regions bound by both GATA4 and p300 (8/9, 88.9%). Table 1 List of selected enhancers tested in the transient transgenic enhancer assay. 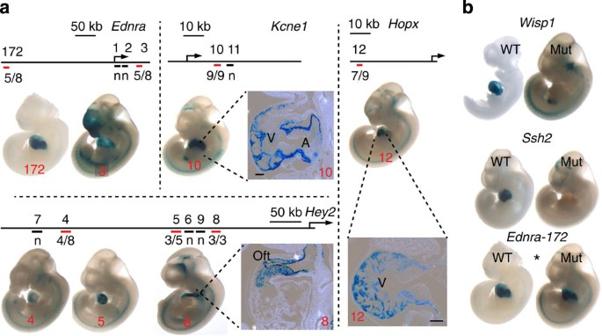Figure 2: Selected GATA4 distal regions tested for enhancer activity in E11.5 transgenic embryos. (a) Enhancer-hsp68-lacZ constructs were used to generate E11.5 transgenic embryos. Red bars denote GATA4 regions with heart enhancer activity, while black bars indicate GATA4 regions without heart enhancer activity. Numbers above line indicate the region ID number shown ina. Numbers below line indicate the number of embryos with heart activity and the total number of transgenic embryos examined. n, negative for activity in heart. (b) GATA motif mutation in GATA4 heart enhancers reduced their transcriptional activity. GATA motif mutation inWisp1andSsh2enhancers ablated cardiac activity. ForEdnra-172, mutation of 4 of 5 GATA motifs did not impair heart activity (*). Full size table Figure 2: Selected GATA4 distal regions tested for enhancer activity in E11.5 transgenic embryos. ( a ) Enhancer-hsp68-lacZ constructs were used to generate E11.5 transgenic embryos. Red bars denote GATA4 regions with heart enhancer activity, while black bars indicate GATA4 regions without heart enhancer activity. Numbers above line indicate the region ID number shown in a . Numbers below line indicate the number of embryos with heart activity and the total number of transgenic embryos examined. n, negative for activity in heart. ( b ) GATA motif mutation in GATA4 heart enhancers reduced their transcriptional activity. GATA motif mutation in Wisp1 and Ssh2 enhancers ablated cardiac activity. For Ednra -172, mutation of 4 of 5 GATA motifs did not impair heart activity (*). Full size image We next asked if GATA4 binding is essential for activity of these GATA4-occupied enhancers. We mutated the consensus GATA4 motifs found under the high confidence GATA4 peaks of three enhancers ( Ednra -172, Wisp1 and Ssh2 ) with heart activity ( Table 1 ). Mutation of the GATA motifs in the Wisp1 and Ssh2 enhancers ablated cardiac enhancer activity ( Fig. 2b ). However, mutation of the GATA motif in Ednra -172 did not ( Fig. 2b ), although the mutated enhancer tested still contained an additional GATA motif with significant GATA4 occupancy by bioChIP-seq. We previously reported on the in vivo GATA4 dependence of a fourth region related to Smarcd3 (ref. 8 ), where mutation of both a GATA4 and a TBX5 motif blocked enhancer activity. In summary, GATA motifs were essential for the heart activity of three of four tested GATA4-bound heart enhancers ( Table 1 ). GATA4 promotes deposition of H3K27ac at distal enhancers Fetal GATA4 predominantly binds to distal transcriptional enhancer sequences that are enriched in p300 occupancy. p300 acetylates histone H3 at lysine 27 (H3K27ac), a major active transcriptional enhancer [15] , [16] mark. We hypothesized that an important mechanism by which GATA4 promotes cardiac gene transcription is through GATA4-dependent H3K27ac deposition. To test this hypothesis, we defined the genome-wide chromatin occupancy of H3K27ac in E12.5 heart ventricle by ChIP-seq. There was extensive overlap between distal H3K27ac and GATA4 chromatin occupancy ( Fig. 3a ), as well as substantial overlap (76.3%) between their associated genes ( Fig. 3b ). Regions bound by both GATA4 and H3K27ac were linked to heart development GO terms (orange bars, Fig. 3c ), while those bound by each factor alone were not. 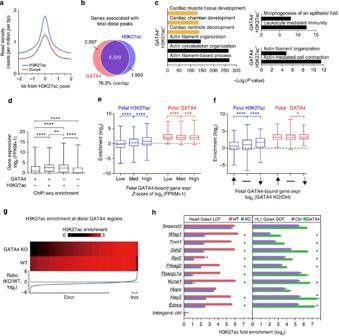Figure 3: GATA4 promotes deposition of H3K27ac at distal regulatory regions. (a) Aggregation plot showing GATA4 enrichment near H3K27ac regions in E12.5 heart ventricle. (b) Overlap of genes associated with fetal distal GATA4 and H3K27ac peaks. (c) GO term analysis of genes associated with distal regions occupied by GATA4 and/or H3K27ac. Orange highlight GO terms related to heart. (d) Box plot shows expression of genes with distal regions occupied by GATA4 and/or H3K27ac. (e) GATA4-bound genes were grouped by their expression level. The peak enrichment of the associated H3K27ac and GATA4 regions was plotted. (f) Genes directly activated by GATA4 were most highly enriched for H3K27ac, and gene expression changes in GATA4 inactivation (GATA4fl/fl::TNT-Cre heart ventricle RNA-seq) correlated with H3K27ac but did not closely correlate with GATA4 binding strength. (g) H3K27ac ChIP-seq was performed in GATA4fl/fland GATA4fl/fl::TNT-Cre heart ventricles. The plot shows H3K27ac signal at distal GATA4 regions, with regions ordered by the ratio of the H3K27ac signal in Gata4 mutant compared with wild type. Decreased or increased H3K27ac was defined as log2(knockout (KO)/wild type (WT))<0.5 or>0.5, respectively. (h) Ten GATA4+H3K27ac+distal regions, one proximal promoter (Smarcd3), and an intergenic control were monitored for H3K27ac enrichment by ChIP quantitative PCR. GATA4 loss-of-function used GATA4fl/fland Gata4fl/fl::TNT-Cre fetal heart ventricle, and gain-of-function used HL1 cardiomyocyte-like cells overexpressing GATA4flbio. Underlined genes were directly activated by GATA4 (Fig. 1c).d–f, Mann–Whitney test;h,t-test. *P<0.05, **P<0.01, ***P<0.001, ****P<0.0001. Error bars show s.e.m. Figure 3: GATA4 promotes deposition of H3K27ac at distal regulatory regions. ( a ) Aggregation plot showing GATA4 enrichment near H3K27ac regions in E12.5 heart ventricle. ( b ) Overlap of genes associated with fetal distal GATA4 and H3K27ac peaks. ( c ) GO term analysis of genes associated with distal regions occupied by GATA4 and/or H3K27ac. Orange highlight GO terms related to heart. ( d ) Box plot shows expression of genes with distal regions occupied by GATA4 and/or H3K27ac. ( e ) GATA4-bound genes were grouped by their expression level. The peak enrichment of the associated H3K27ac and GATA4 regions was plotted. ( f ) Genes directly activated by GATA4 were most highly enriched for H3K27ac, and gene expression changes in GATA4 inactivation (GATA4 fl/fl ::TNT-Cre heart ventricle RNA-seq) correlated with H3K27ac but did not closely correlate with GATA4 binding strength. ( g ) H3K27ac ChIP-seq was performed in GATA4 fl/fl and GATA4 fl/fl ::TNT-Cre heart ventricles. The plot shows H3K27ac signal at distal GATA4 regions, with regions ordered by the ratio of the H3K27ac signal in Gata4 mutant compared with wild type. Decreased or increased H3K27ac was defined as log2(knockout (KO)/wild type (WT))<0.5 or>0.5, respectively. ( h ) Ten GATA4 + H3K27ac + distal regions, one proximal promoter ( Smarcd3 ), and an intergenic control were monitored for H3K27ac enrichment by ChIP quantitative PCR. GATA4 loss-of-function used GATA4 fl/fl and Gata4 fl/fl ::TNT-Cre fetal heart ventricle, and gain-of-function used HL1 cardiomyocyte-like cells overexpressing GATA4 flbio . Underlined genes were directly activated by GATA4 ( Fig. 1c ). d – f , Mann–Whitney test; h , t -test. * P <0.05, ** P <0.01, *** P <0.001, **** P <0.0001. Error bars show s.e.m. Full size image We evaluated the relationship of distal GATA4 or H3K27ac occupancy to the expression of associated genes. The most highly expressed group of genes was associated with distal regions enriched for both GATA4 and H3K27ac ( Fig. 3d ). Genes with distal regions enriched for H3K27ac but not GATA4 were expressed at nearly the same level. In comparison, genes with distal regions enriched for GATA4 but not H3K27ac were expressed at lower levels, and genes with distal regions lacking either feature were the lowest expressed. Increasing expression of GATA4-bound genes correlated with higher H3K27ac enrichment but not with the degree of GATA4 binding ( Fig. 3e ). In fact, fetal heart genes directly activated by GATA4 (bound by GATA4 and downregulated in G4 CKO ) had significantly higher H3K27ac enrichment than genes unaffected or repressed by GATA4 ( Fig. 3f ). In comparison, GATA4 enrichment was not substantially different between genes activated, repressed or unaffected in G4 CKO ( Fig. 3f ). Together, these data indicate that H3K27ac but not GATA4 signal strength associates with higher gene expression. To test the hypothesis that distal GATA4 occupancy promotes H3K27ac deposition, we measured the effect of cardiomyocyte-specific loss of GATA4 on H3K27ac chromatin occupancy ( Fig. 3g ). H3K27ac ChIP-seq on E12.5 G4 CKO or control (Gata4 fl/fl ) heart ventricles demonstrated marked reduction of H3K27ac at 73.3% of fetal distal GATA4 regions, compared with H3K27ac increase at only 5.2% of these regions ( Fig. 3g ; Fisher exact P <8.95E−321). We confirmed this result by preparing chromatin from independent E12.5 G4 CKO or control heart ventricles and measuring H3K27ac enrichment by ChIP quantitative PCR. At 9 of 10 distal fetal GATA4 regions examined, including prospective enhancers of Ppargc1a , Prkag2 , Ryr2 , Tnnt1 , Hey2 and Ednra , GATA4 inactivation significantly reduced H3K27ac enrichment ( Fig. 3h ). On the other hand, GATA4 gain-of-function in HL1 cardiomyocyte-like cells significantly increased H3K27ac enrichment at eight of these regions ( Fig. 3h ). Together, these data show that GATA4 plays a permissive role in gene regulation, but its binding strength as assessed by ChIP-seq does not correlate with the level of gene transcription. Rather, GATA4 stimulates deposition of H3K27ac, which then drives cardiac gene expression. Dynamic changes in GATA4 binding during development To determine changes in GATA4 chromatin occupancy that occur during normal development, we performed GATA4 bioChIP-seq on adult heart ventricles. In biological duplicate samples, we identified greater than 15,000 binding sites, with 13,504 (83.4%) overlapping between replicates. Previously reported GATA4 antibody ChIP-seq from whole adult heart identified less than one seventh the number of GATA4 regions (1,756) [17] , although 69.6% of these overlapped with our bioChIP-seq peaks. By contrast, GATA4 antibody ChIP-seq identified 4409 GATA4 regions in adult fetal liver, [18] and only 22.8% of these regions overlapped our heart ventricle bioChIP-seq peaks. These data suggest that most GATA4 chromatin occupancy is tissue specific. We compared the peaks shared by biological duplicate bioChIP-seq samples from fetal heart with those from adult ( Fig. 4a,b ; Supplementary Fig. 3a ; Supplementary Data 1 ). Of the 13,504 adult GATA4 regions, 8,716 (66.5%) ‘Shared’ regions were reproducibly also occupied by GATA4 in fetal heart. On the other hand, 4,339/13,504 (33.5%) adult GATA4 regions were not bound by GATA4 in fetal heart (‘adult-specific’), and 35,084/43,800 (80.1%) fetal GATA4 regions were not bound by GATA4 in adult heart (‘fetal-specific’). While reduced GATA4 expression in the adult heart ( Supplementary Fig. 3b ) may contribute to the lower number of adult GATA4 regions, this does not account for the ‘adult-specific’ GATA4 regions bound in adult and not fetal heart. 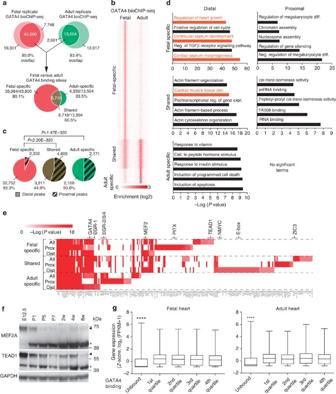Figure 4: Dynamic GATA4 occupancy from fetal to adult heart controls distinct gene programs. (a) Overlap of GATA4 regions between fetal and adult heart. (b) Tag heatmap showing the GATA4 signal intensity at fetal-specific, adult-specific and shared regions (4 kb wide, centred on the GATA4 peak). (c) The genomic distribution of GATA4 regions in fetal and adult heart. P value (Fisher exact test) indicates significance of peak distribution difference. (d) GO term analysis showed that heart-related terms (orange bars) were only enriched in the fetal-specific distal and shared distal regions. (e) TF motifs overrepresented in GATA4-bound regions. The top 1,000 GATA4 regions in the indicated region classes were used forde novomotif discovery. The heatmap displays statistically overrepresented motifs that mapped to JASPAR and TRANSFAC motifs. (f) Downregulation of cardiac TFs MEF2A and TEAD1 during heart development. Arrowhead indicates the full-length protein. Asterisk indicates a smaller immunoreactive band. (g) Box plot of the relationship of GATA4 binding strength to gene expression in fetal and adult stages. GATA4 peaks were ranked by enrichment score and divided into quartiles (first quartile=lowest binding strength). Plot shows expression of genes associated with peaks in each quartile. GATA4-bound genes were more highly expressed than unbound genes, but among bound genes there was no correlation between binding strength and gene expression level. Mann–Whitney test was used for statistical analysis. ****P<0.0001 compared with each other group. Figure 4: Dynamic GATA4 occupancy from fetal to adult heart controls distinct gene programs. ( a ) Overlap of GATA4 regions between fetal and adult heart. ( b ) Tag heatmap showing the GATA4 signal intensity at fetal-specific, adult-specific and shared regions (4 kb wide, centred on the GATA4 peak). ( c ) The genomic distribution of GATA4 regions in fetal and adult heart. P value (Fisher exact test) indicates significance of peak distribution difference. ( d ) GO term analysis showed that heart-related terms (orange bars) were only enriched in the fetal-specific distal and shared distal regions. ( e ) TF motifs overrepresented in GATA4-bound regions. The top 1,000 GATA4 regions in the indicated region classes were used for de novo motif discovery. The heatmap displays statistically overrepresented motifs that mapped to JASPAR and TRANSFAC motifs. ( f ) Downregulation of cardiac TFs MEF2A and TEAD1 during heart development. Arrowhead indicates the full-length protein. Asterisk indicates a smaller immunoreactive band. ( g ) Box plot of the relationship of GATA4 binding strength to gene expression in fetal and adult stages. GATA4 peaks were ranked by enrichment score and divided into quartiles (first quartile=lowest binding strength). Plot shows expression of genes associated with peaks in each quartile. GATA4-bound genes were more highly expressed than unbound genes, but among bound genes there was no correlation between binding strength and gene expression level. Mann–Whitney test was used for statistical analysis. **** P <0.0001 compared with each other group. Full size image Adult and fetal GATA4 regions differed considerably in their location. Around 83.7% of fetal GATA4 regions were distal to TSSs (defined as beyond −2 to +2 kb of the TSS), consistent with our prior findings in the HL1 cardiomyocyte-like cell line [8] . However, adult GATA4 regions shifted markedly towards proximal binding, as only 46.6% were distally located. Similarly, 93.3, 44.9 and 50% of fetal-specific, shared and adult-specific GATA4 regions were distally located, respectively ( Fig. 4c and Supplementary Fig. 3c ). Fetal-specific, shared and adult-specific GATA4 regions were associated with different functional terms ( Fig. 4d and Supplementary Fig. 3d,e ). Distal GATA4 sites that were fetal-specific or shared were associated with GO terms pertaining to heart development (orange bars, Fig. 4d ). Distal fetal-specific GATA4 regions were also linked to ‘positive regulation of cell cycle process’ and ‘regulation of TGFβ receptor signalling pathway’, consistent with GATA4 regulation of cardiomyocyte proliferation [4] , [19] and its interaction with Smad proteins, nuclear targets of TGFβ signalling [20] . Cardiac TFs collaboratively bind to chromatin loci [8] , and changes in GATA4 binding partners might account for altered chromatin occupancy during development [21] , [22] . To identify potential partners, we performed de novo motif discovery on GATA4-bound regions ( Fig. 4e ). As expected, the GATA motif was highly overrepresented in GATA4-bound regions from fetal and adult heart, with adult-specific proximal regions (2,171 regions) being the sole exception. The co-enriched motifs of other TFs were mostly distinct between fetal-specific and adult-specific GATA4-bound regions. For example, the MEF2 motif was strongly enriched in fetal-specific and shared GATA4-bound regions, and the TEAD1 motif was enriched amongst fetal-specific peaks. Shared distal peaks were highly enriched for E-box motifs, which are often bound by bHLH proteins such as HAND1/2 (ref. 23 ). Adult GATA4 regions were highly enriched for the EGR motif, particularly among proximal GATA4 regions. Scanning these regions for the consensus binding motifs for GATA4, MEF2, TEAD1 and EGR1 reinforced these conclusions ( Supplementary Fig. 3f ). These changes in associated motifs might reflect altered expression of transcriptional regulators between fetal and adult heart. For instance, the expression of MEF2A and TEAD1 was significantly lower in adult compared to fetal heart ( Fig. 4f ). We asked if the extent of GATA4 occupancy is related to target gene expression level. GATA4-bound genes were more highly expressed than genes lacking GATA4 binding in both fetal and adult heart ( Fig. 4g ). However, the strength of GATA4 binding did not correlate with gene expression level in either fetal or adult heart. These data are consistent with our analysis of the interplay between GATA4 binding, H3K27ac enrichment and gene expression in the fetal heart, and suggest that this analysis likely also pertains to the adult heart. The chromatin landscape of GATA4-bound regions To further investigate the relationship of GATA4 chromatin occupancy to features of the chromatin landscape, we used ChIP-Seq to establish genome-wide maps of key epigenetic marks (H3K27ac, H3K4me1, H3K27me3 and H3K4me3) and RNA polymerase II (RNAPII) in fetal and adult heart ventricles ( Supplementary Data 1 ). The pattern of these chromatin landscape features at TSSs and at active enhancers (defined by H3K27ac enrichment distal to TSSs; Supplementary Fig. 4a ) was consistent with previous reports [15] , [24] , [25] , [26] , supporting the fidelity of these data. We analysed the aggregate signal for each of these marks centred around fetal and adult GATA4 peaks, each subdivided into locations proximal or distal to TSSs ( Fig. 5a and replicate Supplementary Fig. 4b ). GATA4 peaks were depleted for H3K27me3, a repressive mark. Shared distal and proximal GATA4 regions were enriched for H3K27ac ( Figs 5a v—viii), an activating mark found at enhancers and also present near the TSS [15] . These regions were also enriched for H3K4me3 and RNAPII, activating marks most highly enriched at TSSs (ref. 27 ) and also found at enhancers [28] , [29] . H3K4me1, a mark found at enhancers and to a lesser extent at promoters [30] , also was enriched in the Shared GATA4 regions, with the exception of shared proximal regions of the adult heart. Thus, Shared GATA4-bound regions featured chromatin landscapes rich in activating marks, in both fetal and adult heart. 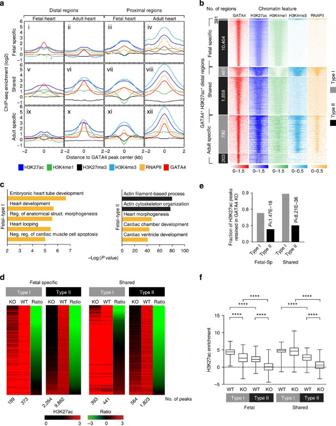Figure 5: The chromatin landscape of GATA4 regions influences their reliance on GATA4 for H3K27ac accumulation. (a) The chromatin landscape at GATA4 proximal and distal regions in the fetal and adult heart. Aggregate curves of ChIP-seq enrichment are plotted centred on GATA4. Arrows inipoint out the lack of enrichment of H3K4me3 and RNAPII, which are found at other enhancers. (b) ChIP-seq tag heat maps are shown for the chromatin landscape feature indicated. The regions are distal fetal-specific or adult-specific GATA4 regions. The regions were groups into those with (type I) and without (type II) H3K4me3 and RNAP2 enrichment. Each region is 2 kb around the peak centre. (c) GO term analysis of genes associated with distal GATA4 regions co-occupied by type I or type II chromatin signatures in fetal heart. Orange bars highlight GO terms related to heart. (d) Change in H3K27ac enrichment of type I versus type II regions with GATA4 loss-of-function. H3K27ac enrichment in Gata4fl/fl::cTNT-Cre or Gata4fl/flcontrol E12.5 heart at distal GATA4 regions is displayed as heat maps. The regions are ordered by the knockout (KO)/wild type (WT) H3K27ac ratio. The number of peaks in each condition is indicated below the heat maps. (e) Plot of the fraction of H3K27ac peaks retained in GATA4 knockout. H3K27ac at type II peaks was more sensitive to GATA4 loss of function. (f) Box plot comparing H3K27ac enrichment in GATA4 knockout or control at distal GATA4 regions with different chromatin environments.e, Fisher exact test.f, Mann–Whitney test. ****P<0.0001. Figure 5: The chromatin landscape of GATA4 regions influences their reliance on GATA4 for H3K27ac accumulation. ( a ) The chromatin landscape at GATA4 proximal and distal regions in the fetal and adult heart. Aggregate curves of ChIP-seq enrichment are plotted centred on GATA4. Arrows in i point out the lack of enrichment of H3K4me3 and RNAPII, which are found at other enhancers. ( b ) ChIP-seq tag heat maps are shown for the chromatin landscape feature indicated. The regions are distal fetal-specific or adult-specific GATA4 regions. The regions were groups into those with (type I) and without (type II) H3K4me3 and RNAP2 enrichment. Each region is 2 kb around the peak centre. ( c ) GO term analysis of genes associated with distal GATA4 regions co-occupied by type I or type II chromatin signatures in fetal heart. Orange bars highlight GO terms related to heart. ( d ) Change in H3K27ac enrichment of type I versus type II regions with GATA4 loss-of-function. H3K27ac enrichment in Gata4 fl/fl ::cTNT-Cre or Gata4 fl/fl control E12.5 heart at distal GATA4 regions is displayed as heat maps. The regions are ordered by the knockout (KO)/wild type (WT) H3K27ac ratio. The number of peaks in each condition is indicated below the heat maps. ( e ) Plot of the fraction of H3K27ac peaks retained in GATA4 knockout. H3K27ac at type II peaks was more sensitive to GATA4 loss of function. ( f ) Box plot comparing H3K27ac enrichment in GATA4 knockout or control at distal GATA4 regions with different chromatin environments. e , Fisher exact test. f , Mann–Whitney test. **** P <0.0001. Full size image We next considered distal, stage-specific GATA4 binding sites ( Fig. 5a , boxes i and x). These were also enriched for H3K27ac, suggesting that many of these regions are functional enhancers. Distal adult-specific GATA4 regions had H3K27ac enrichment in adult but not fetal heart ( Fig. 5a , box x versus ix), suggesting that many of these regions are adult-specific functional enhancers. Consistent with this conclusion, there was also significant H3K4me3 and RNAPII enrichment at the large majority of these sites in adult but not fetal heart. However, a different pattern was observed at distal fetal-specific GATA4 regions—these showed H3K27ac enrichment that was relatively weaker than seen at the adult-specific GATA4 regions, and that was not substantially different between fetal and adult stages ( Fig. 5a , box i versus ii). Furthermore, these fetal distal peaks lacked H3K4me3 and RNAPII (arrows, Fig. 5a , box i). To further investigate the chromatin landscape at GATA4-occupied distal enhancers, we analysed tag heat maps of GATA4 + H3K27ac + distal regions ( Fig. 5b and replicate Supplementary Fig. 4c ). 79.6% of distal adult-specific GATA4 regions displayed a typical enhancer signature (H3K27ac + , H3K4me3 + , RNAPII + ) in the adult heart, which we refer to as type I distal GATA4 regions, whereas 96.4% of distal fetal-specific GATA4 regions displayed the less typical enhancer signature (H3K27ac + , H3K4me3 − , RNAPII − ) in the fetal heart, which we designated type II distal GATA4 regions. Shared GATA4 regions also exhibited predominantly (80.1%) the type II chromatin signature in fetal heart. Interestingly, during development 775 (41.7%) type II regions acquire H3K4me3 and RNAPII to become type I regions, whereas only 1 (<0.1%) type I regions lost H3K4me3 and RNAPII to become type II ( Supplementary Fig. 4d ). As a result, shared GATA4 regions have predominantly (74%) a type I chromatin signature in the adult heart. Together, these data indicate that distal fetal GATA4 regions have a significantly different chromatin signature than adult GATA4 regions (Fisher exact P <0.0001). We examined the biological significance of the type II GATA4 region chromatin signature. To determine if these regions have in vivo heart enhancer activity, we reviewed available in vivo heart enhancer test data. In our enhancer testing and in the VISTA enhancer database [13] , [31] , there were 97 GATA4 + H3K27ac + regions with a type II fetal heart chromatin signature. 66 (68%) had heart activity. Only six regions with a type I fetal heart chromatin signature were tested in the in vivo enhancer assay, and 4 (66%) were positive. Both type I and type II fetal GATA4 regions were overrepresented for GO terms related to heart development ( Fig. 5c ; orange bars). Type II regions were also related to TGF-beta signalling and cell cycle regulation, processes known to be under GATA4 regulation [20] , [32] . These results indicate that a subset of GATA4 + H3K27ac + regions with type I or II signatures are bona fide heart enhancers. We next asked whether enrichment of H3K27ac at fetal distal type I or type II peaks differed in their dependence on GATA4. We analysed our data on H3K27ac occupancy in G4 CKO versus control E12.5 heart ventricle, comparing the change of H3K27ac observed at type I and type II distal fetal-specific and shared GATA4 regions ( Fig. 5d–f ). In control hearts, overall H3K27ac signal was significantly lower at type II compared to type I regions ( Fig. 5f ), and GATA4 inactivation reduced H3K27ac enrichment so that only 23% of type II regions were identified as H3K27ac peaks in mutant hearts ( Fig. 5d,e ). In comparison, 49.3% of type I peaks continued to be identified as H3K27ac peaks in mutants (Fisher P =1.47E−18). The same was true of shared distal regions, where only 31% of type II regions retained H3K27ac in GATA4 knockout, compared with 89.1% of type I regions ( P =8.21E−36). These results indicate that the chromatin landscape of regulatory regions influences their dependence on GATA4 for establishment or maintenance of H3K27ac. Reactivated and new enhancers in adult pressure overload GATA4 plays an integral role in pathological cardiac hypertrophy, in which stress such as pressure overload induces abnormal cardiomyocyte growth and gene expression [1] , [5] . Reactivation of a ‘fetal transcriptional programme’, in which genes normally downregulated between fetal and adult heart are re-expressed in pressure overload, has been described as an integral component of cardiac hypertrophy. While individual examples of fetal gene reactivation are well described, the extent to which the transcriptional circuitry of the fetal heart is redeployed in pathological hypertrophy is unknown. We used RNA-seq to compare cardiac gene expression in mice with pressure overload induced by a surgically placed ligature around the aorta (‘band’) to mice that had undergone sham operation (‘sham’). Out of 1,016 hypertrophic genes ( Supplementary Data 3 ), defined as genes upregulated by more than 0.5-fold (log 2 scale=1.41-fold linear scale) in band, 383 (37.7%) were associated with distal fetal-specific GATA4 regions ( Fig. 6a ). In comparison, only 86 (8.5%), 125 (12.3%) and 204 (20.1%) regions with distal adult-specific, shared and no GATA4 binding were associated with hypertrophic genes, respectively. GO term analysis of the overlapped genes yielded cardiac-related terms in the distal fetal-specific and shared groups (orange bars, Fig. 6a ). In contrast, GO term analysis of hypertrophic genes with adult-specific or no GATA4 binding did not yield functional terms related to the heart. 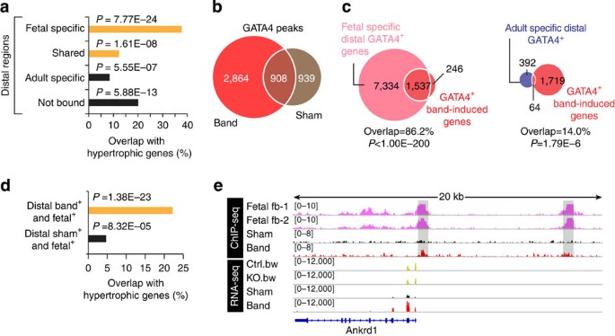Figure 6: GATA4 chromatin occupancy and gene expression changes in pressure overload. (a) Genes upregulated in banding (‘hypertrophic genes’) showed the greatest overlap with genes associated to distal fetal GATA4 peaks. Peaks were mapped to genes (see Methods) and genes were filtered for detectable expression (FPKM>=1). ‘Not bound’ indicates genes without distal GATA4 binding in fetal or adult heart.Pvalue indicates significance of overlap, using the hypergeometric test. (b) GATA4 bioChIP-seq of band and sham heart showing the extent of peak overlap. Peaks include proximal and distal regions. Peaks unique to band were defined as band-induced GATA4 regions. (c) GATA4+band-induced genes, defined as genes associated with distal GATA4 peaks found in band but not sham, overlapped with genes associated with distal fetal GATA4 regions. There was less overlap with genes associated with distal adult GATA4 regions.Pvalue indicates significance of overlap, using the hypergeometric test. (d) Hypertrophic genes overlapped significantly with genes that shared both fetal-specific and band-induced GATA4 regions. These overlapped genes were enriched for heart GO terms (indicated by the orange coloured bar). There was less overlap with genes that shared both fetal-specific and sham-specific GATA4 regions, and the genes in this overlap were not enriched for heart GO terms. (e) Example of bioChIP-seq and RNA-seq (reads per 10 M unique mapped reads) data tracks.Ankrd1was downregulated in fetal heart GATA4 knockout and upregulated in band.Ankrd1was strongly bound by GATA4 at both proximal and distal locations in fetal heart (grey boxes). GATA4 occupancy was lower in sham and increased in band. Figure 6: GATA4 chromatin occupancy and gene expression changes in pressure overload. ( a ) Genes upregulated in banding (‘hypertrophic genes’) showed the greatest overlap with genes associated to distal fetal GATA4 peaks. Peaks were mapped to genes (see Methods) and genes were filtered for detectable expression (FPKM>=1). ‘Not bound’ indicates genes without distal GATA4 binding in fetal or adult heart. P value indicates significance of overlap, using the hypergeometric test. ( b ) GATA4 bioChIP-seq of band and sham heart showing the extent of peak overlap. Peaks include proximal and distal regions. Peaks unique to band were defined as band-induced GATA4 regions. ( c ) GATA4 + band-induced genes, defined as genes associated with distal GATA4 peaks found in band but not sham, overlapped with genes associated with distal fetal GATA4 regions. There was less overlap with genes associated with distal adult GATA4 regions. P value indicates significance of overlap, using the hypergeometric test. ( d ) Hypertrophic genes overlapped significantly with genes that shared both fetal-specific and band-induced GATA4 regions. These overlapped genes were enriched for heart GO terms (indicated by the orange coloured bar). There was less overlap with genes that shared both fetal-specific and sham-specific GATA4 regions, and the genes in this overlap were not enriched for heart GO terms. ( e ) Example of bioChIP-seq and RNA-seq (reads per 10 M unique mapped reads) data tracks. Ankrd1 was downregulated in fetal heart GATA4 knockout and upregulated in band. Ankrd1 was strongly bound by GATA4 at both proximal and distal locations in fetal heart (grey boxes). GATA4 occupancy was lower in sham and increased in band. Full size image Next, we examined GATA4 binding changes induced by pressure overload. GATA4 bioChIP-seq identified 1,847 and 3,772 distal GATA4-occupied regions in sham and band heart, respectively. Only 908 GATA4 regions (49%) were shared between sham and band ( Fig. 6b ), suggesting that GATA4 occupancy significantly changes in heart disease. Distal GATA4 regions identified in band only (‘band-induced’) mapped to 1,783 genes, which we referred to as GATA4 + band-induced genes. Most GATA4 + band-induced genes extensively overlapped (86.2%; P <1.00E−200) with genes associated with distal fetal-specific GATA4 regions ( Fig. 6c ), while the extent of overlap with genes associated with distal adult-specific GATA4 regions was far less (14%; P <1.8E−6). The genes related to distal GATA4 regions that were found in both band-induced and fetal-specific peak sets showed significant overlap with hypertrophy genes ( Fig. 6d ; 22.1%; P =1.38E−23). These overlapped genes were enriched for heart-related GO terms (orange bar, Fig. 6d ). In contrast, the genes associated with sham-specific and fetal-specific distal GATA4 regions overlapped less extensively with hypertrophy genes (4.5%; P =8.32E−05) and these overlapped genes were not enriched for heart-related GO terms. To further investigate how disease- and development-associated changes in GATA4 occupancy relate to one another, we compared GATA4 bioChIP-seq signals from fetal, sham and band samples. Figure 6e shows an illustrative example in which two regions, highly enriched for GATA4 in the fetal heart, are adjacent to Ankrd1 , a gene upregulated in band. In sham-operated adult heart, the bioChIP-seq signal was subthreshold, but returned with banding ( Fig. 6e ). Displaying all distal regions with GATA4 enrichment in band but not sham (band-induced regions), categorized by their overlap with fetal-specific, adult-specific and shared regions, yielded an overview of the relationship of GATA4 chromatin occupancy in development and disease ( Fig. 7a ; Supplementary Data 4 ; Supplementary Fig. 5a,b ). This analysis defined a class of band-induced regions with little GATA4 occupancy in normal fetal or adult heart (‘new’, Fig. 7a ), and three additional classes that overlapped with Fetal-Specific, Adult-Specific, and Shared regions. This ‘New’ category contained the most regions, indicating that cardiac stress induced GATA4 to occupy regions that it does not bind in normal heart development. Among the genes associated with these regions were hypertrophy regulators Tead1 , Fhl1 , Ankrd1 and SWI/SNF core component Smarca2 ( Supplementary Fig. 5a ). Additional band-induced GATA4 peaks represented restored GATA4 binding to fetal-specific peaks at genes such as Zfpm2 ( Fog2 ) and Hdac9 ( Supplementary Fig. 5b ). 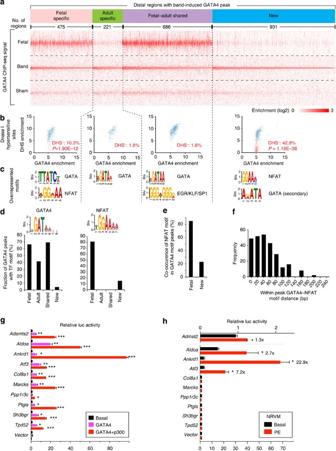Figure 7: The cardiac hypertrophic transcriptional programme reflects re-establishment of fetal GATA4 binding and acquisition of new GATA4 binding sites. (a) Tag heatmap of distal regions containing band-induced GATA4 regions. These regions were classified by their overlap with fetal-specific, adult-specific or fetal-adult shared peaks. Those without overlap were labelled ‘new’. Within each group, regions were sorted by the enrichment score in band. (b) Relationship of band-induced distal GATA4 regions with DNase I hypersensitive sites (DHS) of normal adult heart to GATA4 binding. DHS data were obtained by ENCODE33. Blue and pink indicates regions with and without significant DHS signal, respectively.Pvalue indicates the significance of the difference in overlap of fetal-specific or new regions compared with adult-specific or shared regions (Fisher exact test). (c) Overrepresented motifs found byde novomotif discovery in distal GATA4 band-induced regions, based on their overlap with developmental GATA4 regions. (d) Motif scanning with the indicated motifs showed their frequency in fetal-specific, adult-specific, shared and new classes of distal, band-induced GATA4 regions. (e) Co-occurrence of GATA and NFAT motifs in the same peak region, among distal, band-induced GATA4 regions that overlapped with fetal-specific and new peaks. (f) Distribution of distance of GATA4 and NFAT motifs in the GATA4 peaks ine. (g) Luciferase assay of selected enhancers in 293T cells under basal conditions or in the presence of GATA4 or GATA4+p300 overexpression. (h) Luciferase assay of selected enhancers in neonatal rat ventricular myocytes (NRVMs). NRVMs were transfected with indicated enhancer luciferase constructs and stimulated with or without PE for 30 h. Relative luciferase activity was expressed as fold change against the unstimulated empty vector. Number over bars indicates fold stimulation by PE.b, Fisher exact test.g,h,t-test. *P<0.05; **P<0.01; ***P<0.001. Error bars, s.e.m. Figure 7: The cardiac hypertrophic transcriptional programme reflects re-establishment of fetal GATA4 binding and acquisition of new GATA4 binding sites. ( a ) Tag heatmap of distal regions containing band-induced GATA4 regions. These regions were classified by their overlap with fetal-specific, adult-specific or fetal-adult shared peaks. Those without overlap were labelled ‘new’. Within each group, regions were sorted by the enrichment score in band. ( b ) Relationship of band-induced distal GATA4 regions with DNase I hypersensitive sites (DHS) of normal adult heart to GATA4 binding. DHS data were obtained by ENCODE [33] . Blue and pink indicates regions with and without significant DHS signal, respectively. P value indicates the significance of the difference in overlap of fetal-specific or new regions compared with adult-specific or shared regions (Fisher exact test). ( c ) Overrepresented motifs found by de novo motif discovery in distal GATA4 band-induced regions, based on their overlap with developmental GATA4 regions. ( d ) Motif scanning with the indicated motifs showed their frequency in fetal-specific, adult-specific, shared and new classes of distal, band-induced GATA4 regions. ( e ) Co-occurrence of GATA and NFAT motifs in the same peak region, among distal, band-induced GATA4 regions that overlapped with fetal-specific and new peaks. ( f ) Distribution of distance of GATA4 and NFAT motifs in the GATA4 peaks in e . ( g ) Luciferase assay of selected enhancers in 293T cells under basal conditions or in the presence of GATA4 or GATA4+p300 overexpression. ( h ) Luciferase assay of selected enhancers in neonatal rat ventricular myocytes (NRVMs). NRVMs were transfected with indicated enhancer luciferase constructs and stimulated with or without PE for 30 h. Relative luciferase activity was expressed as fold change against the unstimulated empty vector. Number over bars indicates fold stimulation by PE. b , Fisher exact test. g , h , t -test. * P <0.05; ** P <0.01; *** P <0.001. Error bars, s.e.m. Full size image Most transcriptional regulatory sequences exhibit hypersensitivity to digestion by DNase I (ref. 33 ). To further assess whether these distal GATA4-bound regions likely represent regulatory sequences, we evaluated their DNase I hypersensitivity using publicly data for the normal adult mouse heart [33] ( Fig. 7b ). The large majority (75.4%) of the band-induced GATA4 regions overlapped with DNase I hypersensitive sites (DHSs). Thus, most distal band-induced GATA4 regions had an open chromatin conformation consistent with active transcriptional regulatory regions, and most of these regions already possessed this open signature in the normal adult heart. Interestingly, among the band-induced GATA4 regions that were ‘new’ or reactivated fetal-specific, regions without DHS signal in the normal adult heart were significantly more frequent than in the other two groups ( Fig. 7b ; 42.9% ( P =1.2E−38) and 10.3% ( P =1.90E−12) in new and fetal-specific categories, respectively). These may represent disease transcriptional enhancers recruited as part of the cardiac hypertrophy transcriptional programme. We also analysed GATA4 occupancy of proximal band-induced regions to determine the relationship to GATA4 occupancy in normal fetal and adult heart ( Supplementary Fig. 5c,d ). This genome-wide analysis only yielded 42 (7.6%) and 58 (10.5%) ‘fetal-specific’ and ‘new’ regions, respectively. These sets of regions did not yield any significant GO terms nor were they enriched in known TF motifs. These results indicate that pressure overload does not lead to substantial shift of GATA4 binding to fetal-specific or new proximal regions and that changes in distal rather than proximal GATA4 binding likely play a dominant role in regulation of the hypertrophic response. To identify partner TFs that might drive GATA4 occupancy of distal regions in pressure overload, we performed de novo motif discovery using the four classes of distal, band-induced GATA4 regions ( Fig. 7c ). The distal band-induced peaks that overlapped with GATA4 regions in fetal and/or adult heart were enriched for the consensus GATA motif, while the ‘new’ group of distal band-induced peaks contained an atypical GATA motif. Interestingly, band-induced GATA regions overlapping fetal GATA4 regions, and ‘new’ GATA4 regions, were also enriched for the motif of NFAT ( Fig. 7c ), a calcium-responsive TF family essential for heart development [34] and the heart’s response to pathological stimuli such as pressure overload [35] . Scanning the band-induced peaks for the consensus GATA and NFAT motifs showed that most regions with banding-induced restoration of fetal GATA4 occupancy contained both GATA and NFAT motifs ( Fig. 7d ). Indeed, 85% of the regions with the GATA motif also contained an NFAT motif ( Fig. 7e ), and the motifs were usually located less than 60 bp from each other ( Fig. 7f ). Among the genes relevant to pressure overload hypertrophy that contained GATA4-bound regions with NFAT motifs were Ryr2 , Myocd , Vegfa , Camk2d and the mineraldocorticoid nuclear receptor Nr3c2 ( Supplementary Data 4 ). These data corroborate prior anecdotal data indicative of an important role for NFAT–GATA4 interaction in the cardiac hypertrophic response, and moreover identify candidate enhancers regulated by this interaction. We analysed the functional annotations of genes associated with the band-induced GATA4 regions ( Supplementary Fig. 5e ). Distal band-induced GATA4 regions overlapping shared GATA4 regions were enriched for functional terms related to muscle development and heart contraction, as well as mitochondrial organization. Distal band-induced GATA4 regions overlapping fetal-specific peaks were associated with muscle and artery development, and the subset of these regions that contained both NFAT and GATA motifs was likewise associated with functional terms related to muscle differentiation and cytoskeleton organization ( P <2E−05). To further assess the transcriptional regulatory activity of distal band-induced GATA4 regions, we selected 10 regions linked to genes upregulated in pressure overload. The regions were cloned into luciferase reporter vectors containing basal promoters. Their responsiveness to GATA4 was tested by co-transfection with GATA4 or GATA4 plus p300. GATA4 alone significantly increased transcriptional enhancer activity in 9 of the 10 regions, and introduction of p300 further boosted their activity ( Fig. 7g ). Next, we tested the responsiveness of these regulatory elements to activation of the hypertrophic programme in cardiomyocytes. The enhancer-reporter constructs were transfected into neonatal rat ventricular myocytes treated with the hypertrophic agonist phenylephrine (PE) or vehicle control. PE significantly increased the activity of 4 out of 10 enhancers (1.3–22.9-fold stimulation; Fig. 7h ), whereas 6 enhancers were not detectably stimulated by PE. Testing these adult enhancers in neonatal cardiomyocytes possibly reduced the sensitivity of this assay. Together, these data show that pressure overload activates a hypertrophic programme involving GATA4 recruitment to new disease enhancers that were not occupied by GATA4 during development, as well as restoration of GATA4 binding to a subset of fetal GATA4 enhancers. The dynamic changes in transcription factor chromatin occupancy that occur during development and disease, its relationship to the chromatin environment and its effect on transcriptional regulation, are important incompletely resolved questions. Here, we investigated in depth the chromatin occupancy of the key cardiac transcription factor GATA4 and show that its chromatin occupancy changes dynamically in heart development and disease. We used two independent GATA4 pull-down strategies, streptavidin pull-down of in vivo biotinylated GATA4 and immunoprecipitation, to identify GATA4-bound regions. Establishing a knock in, epitope tagged mouse line is time consuming and resource intensive. The investment in generating the in vivo biotinylated allele proved fruitful, as bioChIP-seq was highly efficient and reproducible and yielded more peaks with higher signal than obtained through antibody-mediated ChIP-seq. Antibody-mediated ChIP-seq remained valuable as an orthogonal method that helped us further hone in on high confidence GATA4-bound regions, but was more variable and far less sensitive. GATA4 chromatin occupancy changed dramatically through development, in concert with its changing function. GATA4 regions in the fetal heart were predominantly distal from TSSs. In adult heart, we observed a dramatic shift of GATA4 regions to TSS proximal locations. Motif analysis indicated that the selection of GATA4 binding sites is influenced by its interactions with TFs: MEF2, TEAD1, and E-box motifs were overrepresented in fetal GATA4 regions, while motifs of EGR1, a TF implicated in regulation of cardiac hypertrophy [36] , were overrepresented in adult GATA4 regions. An important mechanism for GATA4 transcriptional activity was promoting deposition of activating histone marks near its binding sites. Through multiple lines of data, we showed that GATA4 recruits the histone acetyltransferase p300, which deposits H3K27ac deposition at cardiac enhancers to stimulate transcription. These findings provide insights into how TFs such as GATA4 shape the chromatin environment to regulate gene expression. The chromatin landscape of distal GATA4 + H3K27ac + prospective enhancers was different between fetal and adult heart. In adult heart, most of these regions were enriched for RNAPII and H3K4me3, which are commonly found at enhancers [24] , [29] . In contrast, these regions largely lacked RNAPII and H3K4me3 enrichment in fetal heart. Regions lacking RNAPII and H3K4me3 had a greater reliance on GATA4 for their H3K27ac enrichment. One interpretation of these observations is that initially established enhancers lack RNAPII and H3K4me3 enrichment, and in this nascent state require GATA4 to maintain H3K27ac. With time, the enhancers become more well established, accumulate RNAPII and H3K4me3 and reduce their dependence on GATA4 for maintenance of H3K27ac. Additional studies will be required to test these hypotheses and to determine whether these observations are restricted to GATA4 enhancers or are generalizable to other enhancer classes. Pathological stress, such as pressure overload, alters cardiac gene expression and promotes the re-expression of genes predominantly expressed in the fetal heart. This observation has been attributed to reactivation of a fetal gene programme, which implies restoration of TF binding to fetal enhancers. We rigorously tested this model by comparing GATA4 chromatin occupancy in development versus pressure overload. At the gene level, there was a clear relationship between hypertrophic genes and distal fetal GATA4 occupancy patterns. Furthermore, a subset of distal band-induced GATA4 regions did indeed reflect restoration of fetal GATA4 binding. However, reactivation of fetal regulatory regions constitutes a small portion of the transcriptional response of the diseased adult heart. Whereas 20.5% of band-induced GATA4 regions represented re-occupancy of fetal regions, 40.5% were due to GATA4 binding to transcriptional regulatory elements not normally bound by GATA4 in the normal developing or adult heart. These ‘new’ GATA4-bound regions suggest a stress-induced, disease-specific transcriptional programme. Two mechanisms likely contribute to GATA4 recruitment to new distal elements in cardiac hypertrophy. First, the majority of distal elements that overlapped restored fetal binding contained both GATA4 and NFAT motifs. This interaction was previously reported for Nppb and its general significance was inferred from this anecdotal example [35] . Our observation provides unbiased, genome-wide evidence for the importance of GATA4-NFAT co-binding in driving the hypertrophic response and the reactivation of fetal gene expression, and identifies many other enhancers and genes that are likely regulated through this mechanism. Second, we found that 43% of banding-induced GATA4 occupancy of ‘new’ distal sites occurred at sites that have a ‘closed’ chromatin configuration in the normal heart, as assessed by lack of DNase I hypersensitivity. GATA4 has been shown to displace histones from chromatinized DNA. This ‘pioneer’ activity has been proposed to permit GATA4 to initiate formation of transcriptional regulatory complexes on closed chromatin [37] . We propose that GATA4 occupies ‘new’ loci in pressure overload through its pioneer activity. The characteristics that define these ‘new’ loci and their functional significance will be fruitful areas for future study. Mice Gata4 flbio (Jackson Labs, stock #018121) [11] , Rosa26 BirA (Jackson Labs, stock #010920) [38] , cTNT cre [39] and Gata4 flox (Jackson Labs, stock #008194) [6] alleles were described previously. Experiments were performed according to protocols approved by the Institutional Animal Care and Use Committee. Fetal mice were collected at E12.5. Hearts were collected from adult mice at 6–10 weeks of age. The apical half of the heart of fetal and adult hearts was used for chromatin or RNA analysis. Sham and band (ascending aortic band) were performed as described [40] . Hearts were collected 2 weeks after the operation. ChIP and RNA preparation Ventricular apex tissue was used for chromatin and RNA preparation. Both bioChIP and antibody-based ChIP were performed as described [9] . For bioChIP, minced freshly collected tissues were crosslinked with 1% formaldehyde for 15 min at room temperature then terminated with glycine. After PBS rinse, nuclei were isolated by resuspending in Hypotonic Lysis Buffer (20 mM HEPES pH 7.5, 10 mM KCl, 1 mM EDTA, 0.1 mM Na 3 VO 4 , 0.1 mM 0.2% (v/v) Nonidet P40 (NP40), 10% (v/v) glycerol plus protease inhibitor cocktail) and dounce homogenized. Pelleted nuclei were then resuspended in 20 mM Tris (pH 8.0), 2 mM EDTA, 150 mM NaCl, 0.1% SDS, 1% Triton X-100 (TX100) and protease inhibitors. Samples were sonicated, yielding an average fragment size of ~200 bp. After preclearing with Protein G beads, samples were incubated with streptavidin beads (Dynabeads Streptavidin M280) at 4 °C overnight. Beads were washed with a series of buffers containing 2% SDS, 0.1% deoxycholate, 1% T X-100, and high and low salt concentrations. After DNA elution, crosslink reversal and Proteinase K digestion and purification with QIAquick columns (Qiagen), Illumina sequencing libraries were constructed. Antibody-based ChIP was performed as above but without the 2% SDS wash step. ChIP quantitative PCR values were expressed as fold enrichment. Antibodies used were as follows: GATA4, Santa Cruz sc-1237x; H3K4me3, Active Motif 39159; H3K4me1, Abcam ab8895; H3K27ac, Abcam ab4729; H3K27me3, Millipore 17–622; RNAPII, Millipore 17–672. RNA-seq libraries were prepared as described [41] . Briefly, messenger RNA was isolated from total RNA using Dynabeads Oligo(dT), followed by first and second strands synthesis. RNA-seq libraries were prepared from fragmented double-stranded cDNA using ScriptSeq v2 (Epicenter). Transgenic mouse reporter assay Genomic regions covering selected GATA4 regions were amplified and inserted upstream of a minimal hsp68 promoter-LacZ reporter gene as described previously [13] . Transgenic mouse embryos were generated by pronuclear injection. Embryos were collected at E11.5 and stained for LacZ activity as previously described [13] . A region was scored as yielding positive heart activity if three or more transient transgenics from the same construct yielded a reproducible cardiac staining pattern. Luciferase reporter assay Genomic regions were amplified and cloned upstream of a minimal promoter in XhoI and HindIII digested pGL4.23 using the Gibson assembly method. Neonatal rat ventricular myocytes at postnatal day 1 were isolated and co-transfected with pGL4.23-enhancers and phRL-TK with X-tremeGENE HP transfection reagent (Roche), stimulated with or without 100 μM PE for 30 h before the dual luciferase assay. Luciferase activity was normalized to Renilla luciferase activity and expressed as fold change against the empty vector pGL4.23. ChIP-seq data analysis Illumina libraries were sequenced on a Hiseq 2000. Single end 50 nt reads were aligned to mouse reference genome (mm9) using BWA (version 0.5.9) [42] . Reads with no more than 2 bp mismatches and uniquely mapped to reference genome were retained. For duplicated reads with exactly the same genomic coordinates, only one read was kept. Read density was expressed as the number of reads per 10 million uniquely mapped, non-duplicated reads. The peak caller programme MACS (version 1.4) [43] was used to identify peaks with the following parameter settings: --bw=200 --keep-dup=1. We used IGV (version 2.3) [44] or the UCSC Genome Browser to visualize bigwig data tracks. For each track, read number was normalized per 10 million aligned reads. Peaks were assigned to the gene with the closest TSS. Proximal was defined within ±2 kb of the TSS, while remaining regions were defined as distal. Aggregation plots were generated using Homer (version 3.1) [45] . Around 40 kb centred on each peak with 100 bp bin size was used for P300 ChIP-seq data sets, while 4 kb peak region and 10 bp bin size was used for all the other data sets. For heat maps, tag density matrices were calculated using Homer. Around 4 kb centred on each peak with 50 bp bin size was used for Fig. 5b , while 2 kb centred on each peak with 25 bp bin size was used for Fig. 7a . Values plottered were log2 transformed fold enrichment (ChIP signal divided by input signal). Genome regions were associated to the gene with the nearest TSS. RNA-seq analysis Paired-end, 50 nt RNA-Seq reads were mapped to mouse reference genome (mm9) using TopHat (version 1.4.0) [46] with default parameter settings. The mapped reads of each gene were counted by htseq-count (version 0.5.4) [47] with the following parameter setting: -i gene_name -a 20 -s no. Expression levels for each gene were calculated by Fragments Per Kilobase of Transcript (longest transcript of gene) per Million mapped fragments (FPKM). Gene expression value was log2 transformed (FPKM+1) for further analysis. An expressed gene was defined as a gene with FPKM>0 in at least one condition. Differentially expressed genes were identified by a log2 fold change of at least 0.5 Motif analysis De novo motif detection was analysed using DREME [48] with the following parameters: -e 0.00001 -mink 5 -maxk 15. We mapped de novo motifs to a known motif database using TOM TOM [49] with default settings. The Motif database was constructed from MEME suite [50] . Only vertebrate motifs were retained. De novo motifs that did not match known motifs were not used. Motifs with P value<10 −8 identified by DREME and P value<10 −3 identified by TOM TOM were collected for generating the motif heatmap. Motif occurrence within peaks was calculated with FIMO [51] with default parameters for fetal, adult and shared Gata4 peaks and q value<0.5 for band Gata4 peaks. GO analysis The functional enrichment of peak regions for GO terms was performed using GREAT [52] with default parameters. The top 20 terms in the ‘biological process’ section were used. Lists of genes were analysed for GO term enrichment using DAVID [53] . Terms within the top 20 ‘GOTERM_BP_FAT’ category were used. Quantitative PCR and western blotting Real time PCR was used to measure relative ChIP enrichment or gene expression. Quantitative PCR was performed using Sybr green chemistry (VeriQuest master mix; Affymetrix). Primer sequences are listed in Supplementary Data 5 . Western blotting was performed using standard protocols. Full uncropped blots are provided in Supplementary Figs 6 and 7 . Statistical analysis For bar charts, data is presented as mean±s.e.m. For whisker plots, the centre line indicates the median, the box represents the interquartile range, and the whiskers represent the minimum and maximum values. Hypergeometric test was used to assess the significance of overlaps in Venn diagrams. Mann–Whitney test was used to compare box plots. Statistical significance was indicated with: * P <0.05, ** P <0.01, *** P <0.001, **** P <0.0001. Accession codes : The high throughput data used in this study are available through the Cardiovascular Development Consortium Server at https://b2b.hci.utah.edu/gnomex/ . Sign in as guest. The data have also been deposited at GEO, accession number GSE52123 . How to cite this article : He, A. et al. Dynamic GATA4 enhancers shape the chromatin landscape central to heart development and disease. Nat. Commun. 5:4907 doi: 10.1038/ncomms5907 (2014).